Location-specific patterns of exposure to recent pre-pandemic strains of influenza A in southern China Variation in influenza incidence between locations is commonly observed on large spatial scales. It is unclear whether such variation occurs on smaller spatial scales and whether it is the result of heterogeneities in population demographics or more subtle differences in population structure and connectivity. Here we show that significant differences in immunity to influenza A viruses among communities in China are not explained by differences in population demographics. We randomly selected households from five randomly selected locations near Guangzhou, China to answer a questionnaire and provide a blood sample for serological testing against five recently circulating influenza viruses. We find a significant reduction in the frequency of detectable neutralization titers with increasing age, levelling off in older age groups. There are significant differences between locations in age, employment status, vaccination history, household size and housing conditions. However, after adjustment, significant variations in the frequency of detectable neutralization titers persists between locations. These results suggest there are characteristics of communities that drive influenza transmission dynamics apart from individual and household level risk factors, and that such factors have effects independent of strain. There is substantial variation in the timing and incidence of influenza epidemics between populations. During typical non-pandemic influenza seasons in North America, large cities experience seasonal epidemics sooner than rural areas or smaller cities [1] , [2] . A study of pneumonia and influenza incidence in Ontario hospitals from 1992 to 2001 found a significant gradient of decreasing burden of disease from urban to rural populations [3] . This latter finding suggests that the average incidence of influenza over a period of 10 years could be substantially different even between nearby populations. Possible drivers of these differences include heterogeneity in population demographics, climatic variation, differing contact patterns within populations and differences in the connectivity of these populations with others. Differences in timing and incidence could be driven by one or more population characteristics affecting the transmission process. Age is certainly a source of heterogeneity for the rate of transmission and acquisition of influenza [4] . Significant differences in the age distribution between locations could explain variation in rates of infection. However, household size, local vaccine uptake and income are all also known to be associated with influenza incidence [5] , [6] . Population connectivity may also be a driver of differential influenza incidence. During the 2009 H1N1 pandemic, populations with higher rates of travel to Mexico were infected more rapidly than less well-connected populations [7] , [8] , [9] . The timing of peaks of influenza incidence in the pandemic of 1968 has been found to be associated with air travel connectivity between populations [10] . Over smaller scales, correlation of seasonal influenza incidence in US states have been found to be associated with the number of commuters travelling between pairs of states [1] . In addition, differences between regions at large spatial scales in density and seasonality have been shown to affect the evolution of the virus as well as its incidence [11] , [12] . Because of the stochastic nature of transmission, reduced connectivity could drive lower rates of incidence: fewer introductions of influenza to remote populations reduce the number of opportunities for an epidemic to be seeded. However, it is difficult to predict the net impact of low connectivity over a long period of time: each year that passes without a large outbreak will build the number of susceptible individuals for the following years and increase the risk that an outbreak proceeds, when an infectious case is introduced. By comparing influenza incidence between populations and adjusting for individual-level factors known to be associated with influenza transmission, it should be possible to determine whether it is individual level factors or some property of the population (for example, connectivity) that drives variation in incidence. Unfortunately, many influenza infections are mild or asymptomatic, making the direct measurement of influenza incidence challenging. Also, the quality of influenza surveillance can vary markedly even across small geographical areas, making retrospective analysis difficult. Recent analysis of data from assays of animal sera raised against surveillance viral strains has produced self-consistent two-dimensional maps of phenotypic evolution, despite the substantial variability associated with individual assays [13] . Although the multiple influenza infections that humans experience over a lifetime (compared with only single deliberate infections in ferrets) will necessarily make the interpretation of human sera assays more difficult, the success, with which antigenic cartography captures the punctuated drift of inter-pandemic influenza evolution, suggests that there is a role for cross-sectional serological studies of influenza infection. Although variations in antibody titers between populations do not provide definitive proof of variations in incidence, they may be the best evidence available that such differences do exist. Although prospective studies of the particular influenza viruses that circulate in populations through time have been conducted and are ongoing [14] , little has been done to investigate the distribution of immunological profiles in space or time. This study aims to identify variations between locations in the population prevalence of positive influenza antibody response to five recently circulating strains of influenza A, and determine whether these variations can be explained by population characteristics known to be associated with influenza transmission and antibody response. We conducted a household-based cross-sectional serological study of five randomly selected communities in Guangdong, China from July 2009 to September 2009. The five selected communities lie in and around Guangzhou, the provincial capital with more than ten million people. Population density is extremely high (upwards of 1,000 km −2 ) in parts of Guangzhou but relatively low in nearby rural areas. Per capita annual consumption ranges from 21,000 yuan in the urban areas of Guangzhou to 5,200 yuan in the rural areas of Guangdong. The five locations are 46.9, 14.2, 57.6, 59.5, 19.9 km from Guangzhou, respectively. Travel times to the centre of Guangzhou are estimated to be 1.08, 0.52, 1.23, 1.23, 0.63 h, respectively. We tested sera from each of the individuals sampled to determine neutralization (NT) responses to five influenza viruses; three H3N2 viruses (A/Shantou/90/2003 (H3N2), A/Shantou/806/2005 (H3N2), A/Shantou/904/2008 (H3N2)) of the Fujian, Wisconsin and Brisbane clusters, respectively, and two H1N1 viruses (A/Shantou/104/2005 (H1N1) and A/Shantou/92/2009 (H1N1)) of the Solomon Island and Brisbane clusters, respectively. Here we show significant differences in in the frequency of detectable neutralization titers to influenza A viruses above among the five randomly selected communities that is not explained by differences in population demographics alone. Study demographics Of the five study locations, 2 and 5 were closest to Guangzhou and the area of highest density, while locations 1, 3 and 4 were in regions of lower population density ( Fig. 1a ). A total of 273 people consented to participate in the study, 151 of which provided a blood sample for serological testing ( Fig. 1b shows the participant flow). 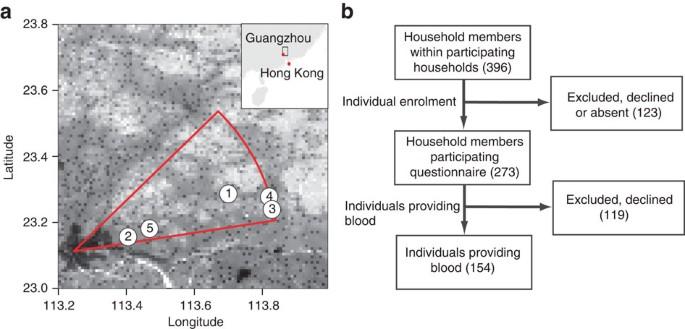Figure 1: Study setup. (a) shows the spatial distribution of study locations and the transect sector from which they were randomly chosen. Greyscale shows population density with darker colours indicating large population density. (b) shows the process of participant recruitment. There were significant differences between study locations for age, years at the address, employment status and vaccination status ( Table 1 ). Study participants in location 5 were younger than in other locations ( Supplementary Fig. S1 ). Overall, self-reported rates of seasonal influenza vaccination were higher than might have been expected for this population (19% vaccinated within the last 5 years versus 1.9% vaccinated per year in all of China) [15] . However, the majority was unvaccinated and many were uncertain whether they had ever been vaccinated. Older individuals were more likely to give blood than younger individuals. Figure 1: Study setup. ( a ) shows the spatial distribution of study locations and the transect sector from which they were randomly chosen. Greyscale shows population density with darker colours indicating large population density. ( b ) shows the process of participant recruitment. Full size image Table 1 Demographic characteristics of study participants. 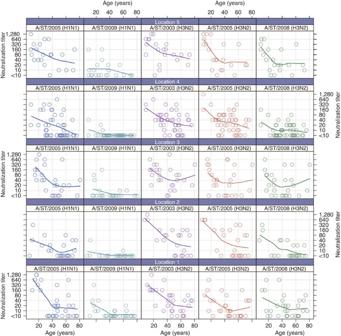Figure 2: Neutralization titers by age and strain, and study location. The line on each chart is a non-parametric local polynomial regression (LOESS) with a span of 0.9 and gaussian distribution family. All charts in the same column show results for the same strain and all charts in the same row show results for the same location. Full size table Similar differences between locations were observed for household-level variables ( Table 2 ). Statistically significant differences were detected between locations within the age structure of households, the area of homes, the proportion with running water, the proportion owning a vehicle and household income. Locations 3 and 4 had more large households (in terms of number of members), whereas household members were less likely to live away from home in locations 1 and 2. Substantial differences between locations were observed for the distribution of sizes of household (in square meters), with location 2 standing out as having only small area households. Location 4 had a much higher proportion of homes without running water than other locations. Table 2 Household characteristics. Full size table Age and detectable neutralization titer Neutralization titers decreased with age for all strains in all locations ( Fig. 2 ). In most cases (location-strain combination), the rate of decrease appears to level off in older ages (between 40 and 60 years of age). In some cases antibody titers appear to increase in the oldest age classes (>60). We compared the running average (20-year width) of percent with detectable neutralization titers (1:10) for each strain, aggregated across locations ( Fig. 3 ). A similar trend was observed to that seen in measured neutralization titers, with a slight uptick in the percentage with detectable titers in the older age groups for the H3N2 strains (A/ST/90/2003 (H3N2), A/ST/806/2005 (H3N2) and A/ST/904/2008 (H3N2)). Using logistic regression, we tested a number of alternative assumptions for the risk of detectable antibodies as a function of age. For all strains other than A/ST/92/2009 (H1N1), models allowing a nonlinear effect of age on the probability of a positive neutralization titer outperformed linear models, with differences in Akaike information criterion (AIC) of 3 or more. Overall, modelling the effect of age using a natural spline with 2 degrees of freedom offered the best fit for the data, as measured by total AIC across strains ( Fig. 3 ), allowing for the levelling off with age seen in the H1N1 strains, and the uptick in the oldest age groups seen in the H3N2 strains. Figure 2: Neutralization titers by age and strain, and study location. The line on each chart is a non-parametric local polynomial regression (LOESS) with a span of 0.9 and gaussian distribution family. All charts in the same column show results for the same strain and all charts in the same row show results for the same location. 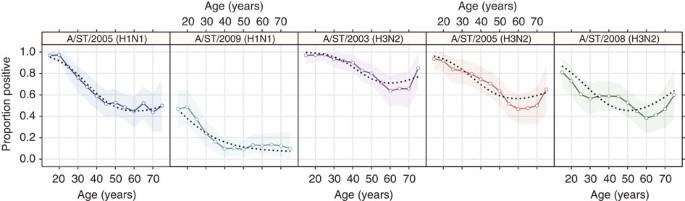Figure 3: Proportion with detectable titers in running 20-year windows by age. Points represent the mid-point of each (overlapping) 20-year age class (point position ±10 years). The shaded regions show bootstrapped 95% confidence intervals (1,000 bootstrap iterations), and blacked dotted lines show the predicted proportion with detectable titers from a logistic-regression on a natural-spline of age with 2 degrees of freedom. Full size image Figure 3: Proportion with detectable titers in running 20-year windows by age. Points represent the mid-point of each (overlapping) 20-year age class (point position ±10 years). The shaded regions show bootstrapped 95% confidence intervals (1,000 bootstrap iterations), and blacked dotted lines show the predicted proportion with detectable titers from a logistic-regression on a natural-spline of age with 2 degrees of freedom. Full size image Location and detectable neutralization titer The overall pattern of neutralization titers shows substantial variation across location and strain ( Fig. 2 ). In Supplementary Table S1 , we show the number (and percent) of samples from each location with detectable levels of titer (>1:10) and present the P value for a χ 2 statistic comparing the detectable titers across locations. Comparison of the percentage of individuals with detectable titers between locations tends to show a consistent pattern regardless of strain ( Fig. 4 ). For instance, the proportion with detectable titers in study site 5 is higher than those in all other study sites, regardless of strain; and, in study site 3, higher titers are seen than in all locations except 5 for the majority of strains (the exception being A/ST/92/2009(H1N1) in comparison to location 1). In most locations, the relative proportion with detectable titers seems to follow a strain-independent pattern, though, for some locations, strain-specific variation appears to exist. For instance, in study site 4, the proportion positive is lower than in study site 1 for all strains other than A/ST/206/2005 (H3N2), for which it is elevated. 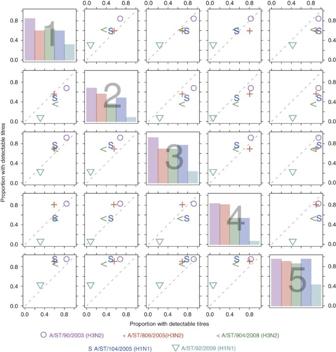Figure 4: Proportions of individuals with detectable neutralization titers across locations. Each point on the off diagonal plots represents the proportion of individuals with detectable titers in the row location (yposition) versus the proportion in the column location (xposition). In the on-diagonal plots, the percentage positive in the indicated location is shown for each strain. Figure 4: Proportions of individuals with detectable neutralization titers across locations. Each point on the off diagonal plots represents the proportion of individuals with detectable titers in the row location ( y position) versus the proportion in the column location ( x position). In the on-diagonal plots, the percentage positive in the indicated location is shown for each strain. Full size image There is a consistent pattern in the proportion positive for individual strains, with A/ST/90/2003 (H3N2) consistently having the highest proportion positive, and A/ST/92/2009 (H1N1) consistently having the lowest proportion positive. Controlling for other covariates by use of conditional logistic regression where each individual represented their own strata of observations, we estimated odds ratios of detecting neutralizing antibody using A/ST/904/2008 (H3N2) as the reference. The odds ratios of detecting neutralizing antibody were estimated to be: A/ST/90/2003 (H3N2) 7.9 (95% CI 3.7, 17.1), A/ST/806/2005 (H3N2) 2.2 (95% CI 1.2, 3.9), A/ST/104/2005 (H1N1) 1.3 (95% CI 0.7, 2.2), A/ST/92/2009 (H1N1) 0.1 (95% CI 0.05, 0.2). Influenza viruses isolated in earlier years were estimated to have higher titer than those isolated later. However, the number of strains we considered is too small to identify a temporal trend. As noted, there are substantial differences between locations in the age distribution of participants. We performed logistic regression of detectable titers on location, adjusting for age to see whether differences in age distribution across location could account for the observed differences in the percentage with detectable titers ( Table 3 ). In the age-adjusted model, we found significant differences from location 1 (reference location) for several strains and locations. In location 2, the probability of detectable neutralization titers was significantly lower for A/ST/904/2008 (H3N2) and A/ST/92/2009 (H1N1). In location 4, the probability of detectable neutralization titers was significantly higher for A/ST/806/2005 (H3N2), and significantly lower for A/ST/92/2009 (H1N1). In location 5, the probability of detecting A/ST/104/2005 (H1N1) was significantly higher. The trend that the probability of detectable titers was more likely in location 5 was maintained in the age-adjusted analysis. Table 3 Log odds ratios of having detectable neutralization titers. Full size table We considered further regression models including individual and household level covariates to see whether these could explain differences between locations and identify other predictors of detectable neutralization titers. A number of models including covariates listed in Tables 1 and 2 were considered ( Table 3 ). Models were compared based on the improvement in fit, as measured by AIC, and whether the extra covariates substantially affected the observed estimates for the effect of location. The best fit model included fever in the past month, location and age as covariates ( Table 3 ), and showed similar significance patterns as the model adjusted only for age. Vaccination was not statistically significantly associated with the probability of detectable titers. The inclusion of housing factors (household area and the presence of running water) showed that, for some strains (A/ST/2003 (H3N2), A/ST/2005 (H3N2) and A/ST/2009 (H1N1)), the presence of running water and large household area (for A/ST/2009 (H1N1)) were significantly associated with detectable neutralization titers and appeared to explain some location differences (perhaps serving as proxies for some unmeasured risk factors). However, the inclusion of these variables did not improve model fit over the age, location and fever model. We fit each of the regression models in Tables 1 and 2 with an additional random effect for household, to account for potential clustering of outcomes within households. We found a very similar pattern of significance among our estimated covariates. The AIC for these models were all higher than the corresponding models that did not include a random effect term. Comparison of neutralization and hemagglutination assays Immunity to each of the strains considered above was also assessed using haemagglutination inhibition (HI) assays. Age-specific patterns in the proportion of individuals with detectable antibody by HI appear qualitatively similar to patterns in detectable antibody by NT. The relative odds of individuals having detectable antibody by strain are nearly identical between HI and NT results. However, there were absolute differences in the proportion of individuals with detectable antibody between the two assays with HI in general, indicating higher rates of positivity. Sensitivity of the results to the cutoff, used to define detectable neutralization titers, was assessed by repeating the regression analyses using cutoffs of 20:1 and 40:1. The use of alternate cutoffs did not qualitatively change the relationships observed, though it did reduce the number of significant results (as would be expected with a less sensitive test). Using a systematic randomization process for spatial location and household, we obtained sera and questionnaire results for 151 individuals in five locations. After adjusting for individual and household level covariates, we found significant differences between locations in the prevalence of detectable neutralization titers to five recently circulating strains of influenza A. We identified a consistent reduction in the frequency of detectable neutralization titers with increasing age, until a threshold is reached at older ages, after which the frequency of detectable titers levels off, or even rises. Multiple mechanisms may create spatial heterogeneity in detectable antibody including intrinsic variation in transmission dynamics or the effect of unmeasured demographic covariates. The observation that each location, in general, shows elevated or decreased detectable antibody across all strains suggests a mechanism that would affect the transmission of all strains. Population density, differing connectivity and differing contact patterns would all be expected to affect the frequency of influenza infection for all strains similarly. Because of logistical constraints, samples were collected sequentially, by location, over a three-month period (July–September). Peaks in influenza incidence in Guangzhou usually occur in July/August and January/February. Recent exposure to influenza has been shown to increase neutralization titers to multiple influenza viruses [16] . The observed differences in neutralization titer by location may be due to sampling occurring at different points in the influenza season. However, the low neutralization titer of A/ST/92/2009(H1N1), a strain known to be circulating locally and contemporaneous with the study, suggests that exposure to this virus was low and the impact of boosting due to exposure to this virus across all strains would be low as well. Van Riet et al found significant differences in responses to influenza immunization in children in rural and urban locations of Gabon [17] . This suggests that factors other than differences in influenza exposure may be responsible for spatial heterogeneity in influenza immunity. However, many of the differences in this population (for example, parasite load) would not be expected to differ in our study population. Although our results suggest that location is a risk factor for influenza exposure, we sampled from only five locations. With this small number, many demographic characteristics of our participants were strongly associated with location, limiting our ability to disentangle the effect on neutralization results of location from the effect of demographic factors. Further locations are needed to determine the specific factors that lead to spatial differences in neutralization patterns. In our findings, age is the factor that most strongly influences the probability of detectable titer. The age-specific pattern of detectable antibody is similar to estimates of age-specific incidence of infection, based on contact models [18] . The age-specific pattern may largely reflect recent exposures with little accumulation of neutralization titers due to cross-neutralizing antibody from multiple exposures to antigenically similar strains. Younger individuals may be more likely to have detectable antibody, because test strains are similar to the strains that first infected these individuals, and responses to antigenically similar viruses yield stronger responses in this case [19] . It is unclear whether the uptick in the frequency of detectable titers among the older age groups for the H3N2 stains is a statistical aberration or represents an actual shift. However, if real, this increase may suggest a more complex pattern of antibody kinetics following infection than previously thought. Confirmation of spatial heterogeneity in influenza immunity in a larger sample may reveal mechanisms that maintain or reduce viral diversity in larger populations. Nonetheless, our study suggests that the exposure of populations to seasonal influenza is heterogeneous at much smaller spatial scales than was previously thought. Containment and mitigation programmes, such as vaccination, may benefit from identifying the causes of spatial variation in influenza transmission and immunity at such scales to target those communities at greatest risk. Selection of study locations Five study locations were selected randomly, with uniform probability across space, from within a study transect. The study transect was a fan-shaped polygon, or sector, with the point of the sector anchored at the location of highest density (as determined by 2008 Landscan data) within Guangzhou ( Fig. 1a ). A radius of 60 km was chosen to balance logistical concerns with our ability to capture a substantial urban–rural gradient. Satellite images for each random location were then reviewed to determine whether the location included at least 20 structures within 1 km of the chosen point. The street or village committee (SVC) that had jurisdiction over the nearest house to the randomly selected location was identified and invited to participate in our study. Locations with less than 20 structures within 1 km or those found to reselect an existing study SVC were rejected and a new location selected. Household recruitment and enrollment of study participants ran from 8 July 2009 until 21 September 2009 ( Fig. 1b ), and, owing to logistical restrictions, the study locations were surveyed and sampled in turn (the sequence of study site visits was: 1, 5, 3, 4, 2). For each study location, a census list of households was obtained from the SVC. From this list, 60 households were randomly selected, and these households were approached in turn. The study team were introduced at the doorstep to households by an SVC member and the household invited to participate. Declining households were not re-approached; invalid addresses were rejected. Members of households agreeing to participate were administered informed consent and offered a choice of two levels of participation: answering an interviewer-led questionnaire on the household and personal information, or completing the questionnaire and providing a blood sample. Households in which no one was present were approached three separate times before discontinuing attempts to contact. Appointments were scheduled with present members of the household to enroll other members not present at the initial household visit. Recruitment continued within each location until 20 households agreed to participate or the sample household list was exhausted. Serological assays HI and virus NT assays were performed for five human seasonal influenza virus strains on each sample of sera: these were strains, isolated locally, that were known to have circulated within Guangdong Province. These strains represent the most frequently detected H3N2 strains in 2003, 2005 and 2008 and the most frequently detected H1N1 strains in 2005 and the early part of 2009 in human surveillance conducted in Guangdong Province. The strains tested were: A/Shantou/90/2003(H3N2), A/Shantou/806/2005(H3N2), A/Shantou/904/2008(H3N2), A/Shantou/104/2005(H1N1) and A/Shantou/92/2009(H1N1). Note that the last strain in the preceding list was not a pandemic virus, but a seasonal H1N1 strain isolated in Guangdong before April 2009. The pandemic virus was not included in our panel because of concern that the timing of sample collection would influence the immunity to the pandemic virus (though little transmission had occurred before testing in all locations). Phylogenetic trees of the H3N2 viruses and H1N1 viruses in relation to vaccine strains of each strain circulating since 1995 are presented in Supplementary Figs S1 and S2 . The 50% tissue culture infectious dose (TCID50) of each stock virus was determined on MDCK (Madin–Darby Canine Kidney) cells. Neutralizing concentrations were defined as the reciprocal of the highest dilution of sera at which 50% of wells were infected, as calculated by the method of Reed and Muench [20] . Sera were thawed and treated with a receptor-destroying enzyme derived from Vibrio cholerae to remove nonspecific inhibitors, then heat-inactivated at 56 °C for 30 min. Before being used in the NT and HI test, receptor-destroying enzyme-pretreated sera were absorbed with Turkey red blood cells to remove substances responsible for nonspecific agglutination. The antibody titer was determined by testing serial twofold dilutions from 1/10 to 1/1,280 in duplicate (uncertain results were resolved by repeating testing in quadruplicate). Positive and negative control sera were also tested and virus back-titration performed. HI assays were conducted in 96-well microtiter plates (Corning Costar) with 0.5% turkey erythrocytes using four hemagglutination units. NT tests were carried out by mixing the serially diluted sera with 100 TCID50 of MDCK cell-adapted viruses of each reference strain, incubated for 1 h at 37 °C and added to a preformed MDCK cell monolayer. Cytopathic effect was read, and heamagglutination assays was performed to detect the presence of virus replication on 3 days post-inoculation. The highest dilution with complete protection of the cell monolayer, in greater than two of the quadruplicate wells, was regarded as the antibody titer. Statistical analysis All statistical analyses were done using the R statistical package (R 2.10, www.cran.org ). Ethics Ethical approval for the study was granted by the Institutional Review Boards of the Johns Hopkins Bloomberg School of Public Health, the University of Hong Kong, the University of Liverpool and Guangzhou Hospital #12. Written consent was obtained from all adult participants (18 or years or older). Children provided verbal assent and their parent or guardian gave written consent. How to cite this article: Lessler, J. et al . Location-specific patterns of exposure to recent pre-pandemic strains of influenza A in southern China. Nat. Commun. 2:423 doi: 10.1038/ncomms1432 (2011).